Constructing chiral bicyclo[3.2.1]octanes via palladium-catalyzed asymmetric tandem Heck/carbonylation desymmetrization of cyclopentenes Transition-metal-catalyzed tandem Heck/carbonylation reaction has emerged as a powerful tool for the synthesis of structurally diverse carbonyl molecules, as well as natural products and pharmaceuticals. However, the asymmetric version was rarely reported, and remains a challenging topic. Herein, we describe a palladium-catalyzed asymmetric tandem Heck/carbonylation desymmetrization of cyclopentenes. Alcohols, phenols and amines are employed as versatile coupling reagents for the construction of multifunctional chiral bicyclo[3.2.1]octanes with one all-carbon quaternary and two tertiary carbon stereogenic centers in high diastereo- and enantioselectivities. This study represents an important progress in both the asymmetric tandem Heck/carbonylation reactions and enantioselective difunctionalization of internal alkenes. Transition-metal (TM)-catalyzed carbonylation reaction [1] , [2] , [3] , [4] , [5] , [6] , [7] , [8] , [9] , [10] , [11] , [12] , [13] , [14] , [15] , [16] , especially palladium-catalyzed tandem Heck/carbonylation reaction, presents an efficient method to construct a variety of synthetically versatile carbonyl compounds from readily accessible organic halides and alkenes [17] , [18] , [19] , [20] , [21] . Moreover, these methods have been applied as key steps in the total synthesis of natural products and bioactive molecules [22] , [23] , [24] , [25] , [26] , [27] , [28] . Very recently, Reisman and co-workers realized the total synthesis of (+)-Perseanol employing palladium-catalyzed tandem Heck/carbonylation to assemble the vital tetracyclic core (Fig. 1a ) [29] . However, the asymmetric version of tandem Heck/carbonylation reactions was rare, and remains a challenging topic. Some inherent issues, such as the strong π-acidity and coordination ability of CO, would hamper the oxidative addition of organohalides towards low-valent metal species [30] . In addition, the harsh reaction conditions (high temperature and high CO pressure), the incidental racemization [31] , the β-hydrogen elimination of alkylpalladium intermediates, the direct carbonylation of organohalides, and other competitive side-reactions make the asymmetric progress more difficult and complicated. Recently, three representative works on palladium-catalyzed asymmetric tandem Heck/carbonylation reaction of 1,1-disubstitueted alkenes to synthesize dihydrobenzofurans, oxindole derivatives, and 3,4-dihydroisoquinolines have been realized by Correia’s group [32] , Zhu and Luo’s group [33] , and Zhang’s group [34] , respectively. In contrast to the success of 1,1-disubstituted alkenes (the alkylpalladium intermediates lack eliminable β-hydrogen), the TM-catalyzed asymmetric tandem Heck/carbonylation reaction of unactivated internal alkenes has not been developed until now. Fig. 1: Palladium-catalyzed tandem Heck/carbonylation reactions of alkenes. a Pd-catalyzed tandem Heck/carbonylation as key step to the total synthesis of (+)-Perseanol. b Palladium-catalyzed asymmetric tandem Heck/carbonylation of internal alkenes towards bicyclo[3.2.1]octanes (this work). c Hypothesis of mechanism for the tandem Heck/carbonylation reaction and foreseeable side reactions. Full size image On the other hand, bicyclo[3.2.1]octanes are found in several natural products with antibacterial, antioxidant, antithrombosis, and antitumor activities [35] , [36] . However, constructing such intricate polycyclic bridge ring compounds with multiple chiral centers simultaneous implementation remains a challenging project [37] , [38] , [39] , [40] , [41] , [42] , [43] , [44] , [45] , [46] . Based on our research interest in Heck reactions [47] , [48] , [49] , [50] , herein, we describe a palladium-catalyzed asymmetric tandem Heck/carbonylation desymmetrization of cyclopentenes to construct multifunctional chiral bicyclo[3.2.1]octanes bearing one all-carbon quaternary and two tertiary carbon stereogenic centers in excellent diastereoselectivities and enantioselectivities (Fig. 1b ). Suppressing the foreseeable side reactions, such as β-hydrogen elimination of alkylpalladium intermediates, and the direct CO insertion or nucleophiles insertion reaction (Fig. 1c ), is the key to the success of this reaction. 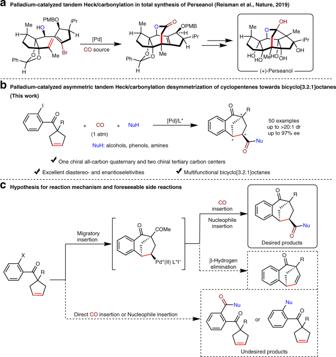Fig. 1: Palladium-catalyzed tandem Heck/carbonylation reactions of alkenes. aPd-catalyzed tandem Heck/carbonylation as key step to the total synthesis of (+)-Perseanol.bPalladium-catalyzed asymmetric tandem Heck/carbonylation of internal alkenes towards bicyclo[3.2.1]octanes (this work).cHypothesis of mechanism for the tandem Heck/carbonylation reaction and foreseeable side reactions. Reaction optimization After systematic evaluation of the reaction conditions, the desired chiral bicyclo[3.2.1]octane product 3aa was achieved in 81% yield and 96% ee employing Pd 2 dba 3 ·CHCl 3 (5 mol%) as the catalyst, ( S )-Difluorphos L1 (20 mol%) as the ligand, K 2 CO 3 (2 equiv) as the base, and mixed 1,2-dichloroethane (DCE)/dichloromethane (DCM) (10/1) as the solvent at 100 °C (Table 1 , entry 1). Other catalysts, such as Pd(OAc) 2 and Pd 2 (dba) 3 were less effective (entries 2 and 3). BINAP L2 , SEGPHOS L3 , DM-SEGPHOS L4 offered 3aa in 52–80% ee (entries 4–6), while BOX-type ligand L5 , PHOX-type ligand L6 , bis(phosphine-amide) ligand L7 and phosphoramidite ligand L8 caused the reaction inactivation (entries 7–10). Decreasing the amount of ligand resulted 3aa in diminished yield, diastereo- and enantioselectivity (entry 11). Screening the additives revealed that K 2 CO 3 was optimal, and AgOAc delivered racemic 3a′ in 83% yield, which was formed via β-hydrogen elimination (entries 1 and 12–14). The choice of solvent, also the ratio of the mixed solvent, was crucial to the reaction efficiency (entries 15–20). Adjusting the reaction temperature was inconducive to improve the outcome of the reaction (entries 21–22). The structure and absolute configuration of 3aa were confirmed by single-crystal X-ray diffraction analysis (see the Supplementary Note 3 for details). Table 1 Optimization of reaction conditions a . Full size table Substrate scope With the optimized reaction conditions in hand, we then tested the substrate scope of alcohols in this asymmetric Heck/carbonylation reaction, and the results were summarized in Fig. 2 . Simple primary alcohols, such as ethanol, n -propanol and benzyl alcohol afforded the products 3aa – ad in moderate to good yields with high enantioselectivities. It is noted that aryl bromine derivative was also a good candidate, delivering 3ab in 50% yield with 94% ee after prolonging the time to 48 h. Besides, other primary alcohols with various functional groups, such as alkenyl, trifluoromethyl, halogen, trimethylsilyl, even highly sterically hindered adamantly group, all performed well, offering 3ae – ai in 88–96% ee. Cyclic and acyclic secondary alcohols delivered the corresponding products 3aj – ao in good efficiency. Products 3ba – da with different substituents on the benzene ring were produced in good yields with high enantioselectivities. Product 3eb with two ester groups was achieved in 68% yield with 95% ee. 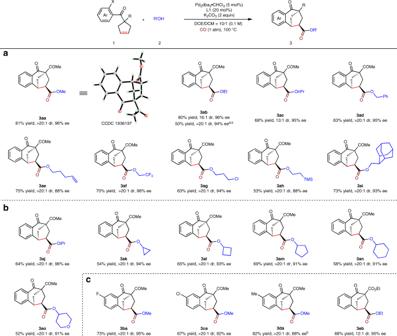Fig. 2: Substrate scope. aSubstrate scope of primary alcohols.bSubstrate scope of secondary alcohols.cSubstrate scope of the benzoylcyclopentenes. Reaction conditions:X= I,1(0.1 mmol),2(1 mmol), Pd2dba3•CHCl3(5 mol%),L1(20 mol%), K2CO3(0.2 mmol) in 1 mL solvent, 100 °C, 36 h, under CO (1 atm). Yields of isolated products are given. The dr values were determined by1H NMR analysis. The ee values were determined by HPLC analysis on a chiral stationary phase.aX = Br.b48 h. Fig. 2: Substrate scope. a Substrate scope of primary alcohols. b Substrate scope of secondary alcohols. c Substrate scope of the benzoylcyclopentenes. Reaction conditions: X = I, 1 (0.1 mmol), 2 (1 mmol), Pd 2 dba 3 •CHCl 3 (5 mol%), L1 (20 mol%), K 2 CO 3 (0.2 mmol) in 1 mL solvent, 100 °C, 36 h, under CO (1 atm). Yields of isolated products are given. The dr values were determined by 1 H NMR analysis. The ee values were determined by HPLC analysis on a chiral stationary phase. a X = Br. b 48 h. Full size image Phenol esters are important skeletons in pharmaceuticals and bioactive compounds. Although phenols as nucleophilic reagents have been employed in some carbonylation reactions [51] , [52] , they have not met with the success in asymmetric tandem Heck/carbonylation reactions, because the two potential nucleophilic sites at O and C of phenols would increase the complexity of the reaction. Herein, phenols as versatile components were performed in our asymmetric Heck/carbonylation reactions with KHCO 3 as the base and toluene as the solvent (Fig. 3 ). Electron donating groups (−Me, − t Bu, and −OMe), a halogen group (−Cl), an electron withdrawing group (−COMe), as well as a phenyl group at the para -position of phenols offered the corresponding products 5aa – ag in 91–95% ee. meta -Chlorine substituted phenol 4h and 3,5-dimethylphenol 4i could also fulfill the reaction well, and no significant steric hindrance effect was observed. 1-Naphthol delivered 5aj in 95% ee. Moreover, monobenzone, as a potent skin lightener drug, could give the adduct 5ak in 91% ee. Fig. 3: Substrate scope of phenols. Reaction conditions: 1a (0.1 mmol), 4 (0.25 mmol), Pd 2 dba 3 •CHCl 3 (5 mol%), L1 (20 mol%), KHCO 3 (0.2 mmol) in toluene (1 mL), 100 °C, 36 h, under CO (1 atm). Yields of isolated products are given. The dr values were determined by 1 H NMR analysis. The ee values were determined by HPLC analysis on a chiral stationary phase. Full size image To further exhibit the robustness and generality of this reaction, scope of nitrogen nucleophiles was investigated with Pddba 2 (10 mol%) as the catalyst, L1 (20 mol%) as the ligand, K 2 HPO 4 (0.2 mmol) as the base in CH 3 CN (1 mL) at 100 °C (Fig. 4 ). Acyclic secondary alkylamines, such as diethylamine and dibenzylamine delivered products 7aa (see the Supplementary Note 4 for details on the X-ray crystal structure) and 7ab in 93 and 94% ee. Cyclic secondary alkylamines furnished products 7ac – ag in 92–94% ee. Alkylarylamines, such as N -methylaniline and indoline, provided 7ah and 7ai in 92 and 91% ee. Primary alkylamines, such as n -propylamine, benzylamines, and thiophenylmethanamine offered products 7aj – am in 92 – 94% ee. Primary arylamines were also qualified to work in this reaction, delivering products 7an – ap in good enantioselectivities with KHCO 3 as the base after prolonging the reaction time to 48 h. 5-OMe-substituted cyclopentene 1f performed smoothly to give 7fb in 97% ee. Finally, pharmaceuticals including Vortioxetine, Trimetazidine and Riluzole were all well late-stage functionalized with bicyclo[3.2.1]octanes to offer 7aq – as in 88–95% ee. Fig. 4: Substrate scope. a Substrate scope of amines. b Application to asymmetric late-stage functionalization of pharmaceuticals. Reaction conditions: 1a (0.1 mmol), 6 (0.2 mmol), Pddba 2 (10 mol%), L1 (20 mol%), K 2 HPO 4 (0.2 mmol) in CH 3 CN (1 mL), 100 °C, 36 h, under CO (1 atm). Yields of isolated products are given. The dr values were determined by 1 H NMR analysis. The ee values were determined by HPLC analysis on a chiral stationary phase. a K 2 HPO 4 was replaced by KHCO 3 , 48 h. b 48 h. Full size image Further study The enantiodivergent synthesis of (5 R , 6 S , 8 S )- 5ac′ was also realized in 70% yield and 97% ee employing ( R )-Difluorphos as the ligand (Fig. 5a ). To demonstrate the mechanism of this reaction, study on nonlinear effect of the enantioselectivity of 5ac was carried out (Fig. 5b ). The linear correlation ( R 2 = 0.99) between the enantioselectivities of the product 5ac and the enantiopurities of the ligand L1 revealed the involvement of one active catalyst species in the stereo-determining transition states of the migratory insertion process. On the basis of the above-mentioned results and previous literatures [31] , [32] , [47] , a proposed mechanism of this reaction is figured in Fig. 5c . 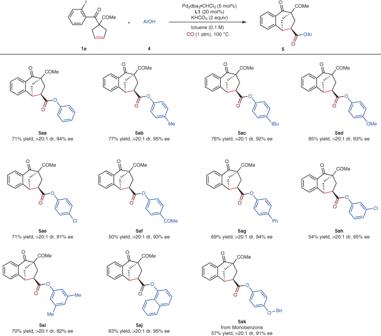Fig. 3: Substrate scope of phenols. Reaction conditions:1a(0.1 mmol),4(0.25 mmol), Pd2dba3•CHCl3(5 mol%),L1(20 mol%), KHCO3(0.2 mmol) in toluene (1 mL), 100 °C, 36 h, under CO (1 atm). Yields of isolated products are given. The dr values were determined by1H NMR analysis. The ee values were determined by HPLC analysis on a chiral stationary phase. Firstly, oxidative addition of the active palladium catalyst with 1a delivers the cationic Pd(II) intermediate I . Intramolecular syn -migratory insertion of I results in the alkylpalladium intermediate II , which followed by the insertion of CO delivers the intermediate III . Finally, the nucleophile insertion of the phenol 4c to the intermediate III produces the product 5ac . It is noted that the high diastereoselectivity was arisen from the stereospecific syn -migratory insertion step, which has been confirmed in our previous work by the deuterium-labeling experiments [47] . The observed stereochemical outcome of the reaction with the C2-symmetric, ( S )-configured ligand L1 can be rationalized based on the two diastereomeric intermediates A1 and B1 (Fig. 5d ). The transition state B1 is notable for the severe steric repulsion between the benzoyl moiety of the cyclopentene 1a and the benzene ring of the ligand L1 , a factor which is not present in the transition state A1 ; this may account for the predominance of the (5 S , 6 R , 8 R ) enantiomer of 5ac in the product. Fig. 5: Further study on the reaction. a Enantiodivergent synthesis of (5 R , 6 S , 8 S )- 5ac′ . b Linear correlation between the ee values of 5ac and L1 . 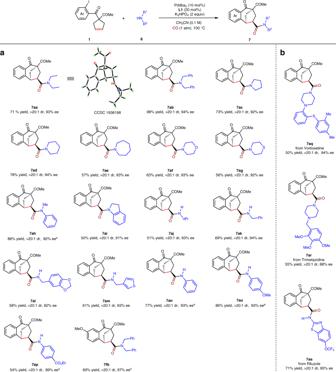Fig. 4: Substrate scope. aSubstrate scope of amines.bApplication to asymmetric late-stage functionalization of pharmaceuticals. Reaction conditions:1a(0.1 mmol),6(0.2 mmol), Pddba2(10 mol%),L1(20 mol%), K2HPO4(0.2 mmol) in CH3CN (1 mL), 100 °C, 36 h, under CO (1 atm). Yields of isolated products are given. The dr values were determined by1H NMR analysis. The ee values were determined by HPLC analysis on a chiral stationary phase.aK2HPO4was replaced by KHCO3, 48 h.b48 h. 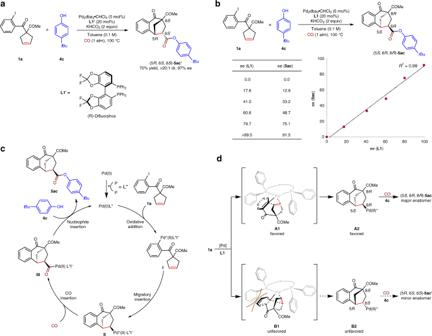Fig. 5: Further study on the reaction. aEnantiodivergent synthesis of (5R, 6S, 8S)-5ac′.bLinear correlation between the ee values of5acandL1.cProposed mechanism.dModel for enantioselectivity. c Proposed mechanism. d Model for enantioselectivity. Full size image In summary, we have developed a Pd-catalyzed asymmetric tandem Heck/carbonylation desymmetrization of cyclopentenes. Various bicyclo[3.2.1]octanes bearing one chiral all-carbon quaternary and two tertiary carbon stereogenic centers were obtained in moderate to good yields with excellent diastereoselectivities and enantiomeric excess. This method provided a general and practical route for the enantioselective difunctionalization of unactivated internal alkenes and chiral bicyclo[3.2.1]octanes. General procedure for the catalytic reactions with alchohols A sealed tube was charged with the cyclopentenes 1 (0.1 mmol, 1 equiv), Pd 2 dba 3 •CHCl 3 (5 mol%), L1 (20 mol%), and K 2 CO 3 (0.2 mmol, 2 equiv). The vial was thoroughly flushed with CO, and alchohols 2 (1 mmol, 10 equiv), as well as DCE/DCM (10/1, 1 mL) were added under CO atmosphere. The reaction mixture was stirred at 100 °C for 36 h. After the reaction vessel was cooled to room temperature, the solution was concentrated in vacuo and purified by careful chromatography on silica gel (200–300 mesh) (PE/EA = 4/1) to afford the desired products 3 . General procedure for the catalytic reactions with phenols A sealed tube was charged with the cyclopentenes 1 (0.1 mmol, 1 equiv), phenols 4 (0.25 mmol, 2.5 equiv), Pd 2 dba 3 •CHCl 3 (5 mol%), L1 (20 mol%), and KHCO 3 (0.2 mmol, 2 equiv). The vial was thoroughly flushed with CO, and toluene (1 mL) was added under CO atmosphere. The reaction mixture was stirred at 100 °C for 36 h. After the reaction vessel was cooled to room temperature, the solution was concentrated in vacuo and purified by careful chromatography on silica gel (200–300 mesh) (PE/EA = 4/1) to afford the desired products 5 . General procedure for the catalytic reactions with amines A sealed tube was charged with the cyclopentenes 1 (0.1 mmol, 1 equiv), Pddba 2 (10 mol%), L1 (20 mol%), and K 2 HPO 4 (0.2 mmol, 2 equiv). The vial was thoroughly flushed with CO, and amines 6 (0.2 mmol, 2 equiv), as well as CH 3 CN (1 mL) were added under CO atmosphere. The reaction mixture was stirred at 100 °C for 36 h. After the reaction vessel was cooled to room temperature, the solution was concentrated in vacuo and purified by careful chromatography on silica gel (200–300 mesh) (PE/EA = 2/1) to afford the desired products 7 .